Activating mutations ofSTAT5BandSTAT3in lymphomas derived from γδ-T or NK cells Lymphomas arising from NK or γδ-T cells are very aggressive diseases and little is known regarding their pathogenesis. Here we report frequent activating mutations of STAT3 and STAT5B in NK/T-cell lymphomas ( n =51), γδ-T-cell lymphomas ( n =43) and their cell lines ( n =9) through next generation and/or Sanger sequencing. STAT5B N642H is particularly frequent in all forms of γδ-T-cell lymphomas. STAT3 and STAT5B mutations are associated with increased phosphorylated protein and a growth advantage to transduced cell lines or normal NK cells. Growth-promoting activity of the mutants can be partially inhibited by a JAK1/2 inhibitor. Molecular modelling and surface plasmon resonance measurements of the N642H mutant indicate a marked increase in binding affinity of the phosphotyrosine-Y699 with the mutant histidine. This is associated with the prolonged persistence of the mutant phosphoSTAT5B and marked increase of binding to target sites. Our findings suggest that JAK-STAT pathway inhibition may represent a therapeutic strategy. Mature NK-cell lymphomas are mostly classified as extranodal NK/T-cell lymphomas of nasal type (NKTCLs) [1] in the World Health Organization classification. 70–90% of NKTCLs are of NK cell lineage with the rest of T-cell origin, most of which are of the γδ type. In current clinical practice, the cases are often lumped together as NKTCL because of similar clinicopathological features and management. NKTCL has poor prognosis, particularly in advanced stage or with extranasal presentation [2] . In this study, we investigate the genome-wide driver mutations in NKTCLs using a combination of RNA sequencing,whole-exome sequencing (WES) and Sanger sequencing, and identify activating mutations of STAT3 and STAT5B in the Src homology 2 (SH2) domain. These mutations are also present at a high frequency (34.9%) in γδ-T-cell-derived lymphomas (γδ-PTCLs) and associated with promotion of growth, which can be partially inhibited by JAK1/2 inhibitors, suggesting a potential therapeutic option for these patients. To identify driver mutations of NKTCLs, whole-transcriptome sequencing (WTS), exome sequencing or targeted Sanger sequencing was applied on 53 NKTCL cases ( Fig. 1a ). 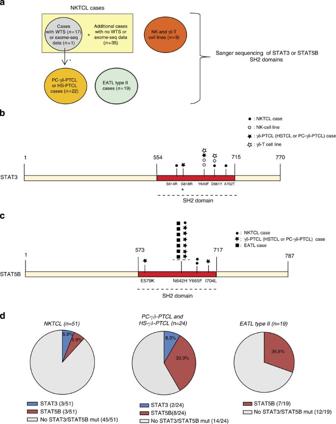Figure 1: Activating STAT3 and STAT5B mutations are frequent in lymphomas of NK or γδ-T cell of origin. (a) The diagram shows the type of mutation analyses performed and the number of tumour samples used for each analysis. The locations of the primers used for PCR and Sanger sequencing of theSTAT3andSTAT5BSH2 domains are shown inSupplementary Fig. 1. The location of the mutated nucleotides found in the SH2 domains ofSTAT3(b) andSTAT5B(c) in tumour cases (NKTCL, γδ-PTCL (PC-γδ-PTCL and HS-γδ-PTCL) or EATL type II) and cell lines (NK and γδ-T cell lines) are shown (not to scale). Mutations of different tumour cases or cell lines are indicated with different symbols over the SH2 domains, and the disease types to which these symbols refer are shown in the upper right corner of the panels. Other than A702T, allSTAT3mutations were reported in LGLL by Koskelaet al.27and Jerezet al.26STAT5B N642H and Y665F mutations were rarely (~1%) observed in LGLL by Rajalaet al.28(d) The percentages of STAT3 and STAT5B mutations in NKTCL (n=51), γδ-PTCL (n=24) or EATL type II cases (n=19) are shown with piecharts. Apart from the STAT5B Y665F mutation identified using WES, all SNVs identified in this study have been cross-validated on genomic DNA with Sanger sequencing using both forward and reverse primers. *: two NKTCL tumour samples with WTS data was re-classified later as PC-γδ-PTCL due to γδ-TCR expression. One of these two reclassified cases is the sample with the STAT3-G618R mutation. First, we validated the mutations detected from our WTS data that may be functionally significant including the mutations in FAS , TP53 , BRAF , MAP2K1 , CREBBP , EP300 and MLL2 genes, by Sanger sequencing on the corresponding genomic DNA ( Supplementary Table 1 ). Of note, FAS and TP53 mutations were identified in NKTCLs by traditional Sanger sequencing in previous studies [3] , [4] . WTS on 17 cases revealed one STAT3 missense single-nucleotide variant (SNV) (S614R, G618R and A702T) in each of three cases (3 of 17, 18%) ( Fig. 1b ). A STAT5B missense mutation (N642H) was present in 1 of the 17 (6%) cases ( Fig. 1c ) and a STAT5B Y665F mutation was identified in a WES analysis on a separate paired NKTCL/normal case. Interestingly, all of the STAT3 and STAT5B SNVs were located in the SH2 domain, a domain critical for STAT activation [5] . Figure 1: Activating STAT3 and STAT5B mutations are frequent in lymphomas of NK or γδ-T cell of origin. ( a ) The diagram shows the type of mutation analyses performed and the number of tumour samples used for each analysis. The locations of the primers used for PCR and Sanger sequencing of the STAT3 and STAT5B SH2 domains are shown in Supplementary Fig. 1 . The location of the mutated nucleotides found in the SH2 domains of STAT3 ( b ) and STAT5B ( c ) in tumour cases (NKTCL, γδ-PTCL (PC-γδ-PTCL and HS-γδ-PTCL) or EATL type II) and cell lines (NK and γδ-T cell lines) are shown (not to scale). Mutations of different tumour cases or cell lines are indicated with different symbols over the SH2 domains, and the disease types to which these symbols refer are shown in the upper right corner of the panels. Other than A702T, all STAT3 mutations were reported in LGLL by Koskela et al . [27] and Jerez et al . [26] STAT5B N642H and Y665F mutations were rarely (~1%) observed in LGLL by Rajala et al . [28] ( d ) The percentages of STAT3 and STAT5B mutations in NKTCL ( n =51), γδ-PTCL ( n =24) or EATL type II cases ( n =19) are shown with piecharts. Apart from the STAT5B Y665F mutation identified using WES, all SNVs identified in this study have been cross-validated on genomic DNA with Sanger sequencing using both forward and reverse primers. *: two NKTCL tumour samples with WTS data was re-classified later as PC-γδ-PTCL due to γδ-TCR expression. One of these two reclassified cases is the sample with the STAT3-G618R mutation. Full size image Because all observed SNVs were located in the SH2 domain, we sequenced the SH2 domains of STAT3 and STAT5B in additional cases. Sanger sequencing of 35 additional NKTCL cases showed a STAT3 D661Y mutation and two STAT5B mutations (Y665F and N642H) in three of these 35 screened cases ( Fig. 1b,c ). These analyses yielded a STAT3 and STAT5B mutation frequency of 5.9% in all NKTCL patients screened by WTS, WES and/or Sanger sequencing ( Fig. 1d , left). RNA-Seq analysis on three NK cell lines revealed an activating mutation, Y640F, in the SH2 domain of STAT3 in NKYS cells, which was validated by Sanger sequencing ( Fig. 1b ). Interestingly, two out of three additional NK cell lines (SNK6 and YT) showed STAT3 mutations when screened by Sanger sequencing, raising the STAT3 mutation frequency to 50% of the six NK cell lines studied ( Fig. 1b ). However, Sanger sequencing of the SH2 domain (ex14–ex18) of STAT5B in these NK cell lines ( Supplementary Fig. 1 ) did not reveal any STAT5B mutations. Two recent studies reported the presence of JAK3 A572V, A573V or V722I mutations in NKTCLs [6] , [7] . However, neither WTS nor hotspot sequencing of 40 NKTCL cases revealed these SNVs, consistent with a recent report [8] . The discrepancy may be due to a variety of factors including the genetic composition of the populations and different stimuli that initiate and sustain the initial phase of NK cell proliferation. Our gene expression profiling studies found that NKTCL and γδ-PTCL cases share a very similar profile with each other and with normal NK cells [9] , suggesting that these two diseases share many functional pathways and may use similar oncogenic mechanisms. Thus, we screened the SH2 domains of STAT3 and STAT5B in 3 γδ-T cell lines and 24 γδ-PTCL cases (15 primary cutaneous (PC)-γδ-PTCL and 9 hepatosplenic (HS)-γδ-PTCL cases). Among the three γδ-T cell lines, we observed a STAT3 Y640F mutation (SNT15) and a STAT3 D661Y mutation (SNT-8), but no STAT5B mutation was observed ( Fig. 1b ). We identified only a STAT3 Y640F mutation in 1 of the 24 γδ-PTCL cases ( Fig. 1b ). On the other hand, 8 of 24 (33.3%) cases (four PC and four HS) showed activating STAT5B mutations in the SH2 domain ( Fig. 1c,d ). Enteropathy associated T-cell lymphoma (EATL) is an aggressive PTCL with higher incidence in the Europe and USA [10] . The disease is now classified into two subtypes: type I is the classical type with TCR-αβ and is associated with celiac disease and gluten-sensitive enteropathy. EATL type II cases have been shown to frequently express TCR-γδ (~78% in one study [11] ), and they are not associated with gluten-sensitive enteropathy. We examined the possibility that STAT3/STAT5B SH2 domain mutations may play a role in EATL type II pathogenesis and identified STAT5B N642H mutations in 7 of 19 cases (36.8%) ( Fig. 1c,d ). Intriguingly, all mutated EATL type II cases have γδ-T-cell receptor expression (7/16 of TCR-γδ-positive cases) underscoring the significance of STAT5B mutations in the neoplastic transformation of γδ-T cells giving rise to different subtypes of γδ-PTCL. To address whether STAT3 mutations activate the STAT3 pathway, we performed western blotting on six NK cell lines using STAT3 and phospho-STAT3 (Tyr705) antibodies. High pY705-STAT3 expression was seen only in mutant cell lines ( Fig. 2a ), suggesting that STAT3 is persistently active in the presence of activating mutations in the SH2 domain. Next, we transduced the NKYS and YT cell lines, which have the activating STAT3-Y640F mutation, with empty vector (EV) or STAT3 shRNA with confirmed activity ( Supplementary Fig. 2a,b ) to evaluate whether STAT3 silencing inhibits the growth of NK cells. We quantified the percentage of GFP positivity of STAT3 shRNA transduced cells at regular time intervals starting 3 days post transduction, and observed a markedly reduced percentage of GFP + cells compared with vector-only transduced cells, suggesting a strong negative selection pressure after STAT3 knock-down ( Fig. 2b–e ). We did not observe a decrease in the percentage of GFP + population in STAT3 shRNA transduced KAI3 cells, which express wild-type (WT) STAT3 ( Fig. 2f,g ). STAT3 protein knock-down efficiency was ~72%, ~78% and ~39% in NKYS, KAI3 and YT cell lines, respectively ( Fig. 2h,i ), which may account for the moderate decrease in growth observed in YT cells after STAT3 knock-down. 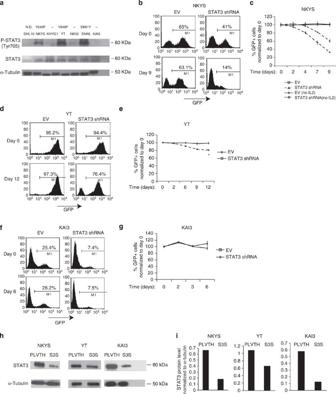Figure 2: NK cell lines with STAT3 mutations show high pY-STAT3 expression and shRNA-mediated knock-down of STAT3 inhibits NK-cell line growth. (a) Western blotting was performed on whole-cell lysates (WCL) from six NK cell lines using antibodies to phosphotyrosine (Y705)-STAT3 and STAT3. DHL16 cells, which lack STAT3 activation, were used as a negative control. α-Tubulin was used as a control to ensure equal loading of the samples. The names of the cell lines used are indicated above the gel image. The type of the corresponding STAT3 mutation is indicated above the name of the cell lines. (−): No STAT3 mutation; N.D., not determined. (b) Representative flow cytometric plots showing the percentage of GFP+cells 3 days (day 0) and 12 days (day 9) post transduction of NKYS cells with EV or STAT3 shRNA after removing IL2 from the culture medium at day 0. (c) Quantification of the percentage of GFP+cells post transduction of NKYS cells with EV or STAT3 shRNA at regular time intervals. In one experiment, cells were cultured in the presence of IL2 (5–7 ng ml−1) until 3 days (day 0) post transduction and then IL2 was removed from the culture medium. In the second experiment, IL2 was always included post transduction of NKYS cells. Each data point is representative of two biological replicates. (d) Representative FACS plots showing the percentage of GFP+cells of YT cell line transduced with EV or STAT3 shRNA 3 days (day 0) or 15 days (day 12) post transduction. (e) Quantification of the percentage of GFP+cells by FACS between 3 and 15 days post transduction with EV or STAT3 shRNA. For 1 week before transduction, YT cells were cultured in the presence of IL2. Three days post transduction (day 0), cells were transferred to medium lacking IL2. *:P<0.05, Student’st-test. (f) Representative FACS plots showing the percentage of GFP+cells in EV or STAT3 shRNA transduced KAI3 cells. (g) Quantification of the percentage of GFP+cells after transduction of KAI3 cells with EV or STAT3 shRNA. Three days post transduction (day 0), the percentage of GFP+cells was determined by flow cytometry, and cells were switched to NK culture medium with reduced IL2 (25 IU ml−1). Data represent means ±s.d. of two biological replicates for panelsc,eandg. (h) Western blot images of STAT3 knock-down levels are shown for NKYS,YT and KAI3 cell lines on STAT3 shRNA transduced, GFP+sorted cells post transduction with the EV (PLVTH) or STAT3 shRNA (S3S). (i) Quantification of the STAT3 protein knock-down levels after normalization to α-Tubulin using the ImageJ program (http://rsb.info.nih.gov/ij/). Figure 2: NK cell lines with STAT3 mutations show high pY-STAT3 expression and shRNA-mediated knock-down of STAT3 inhibits NK-cell line growth. ( a ) Western blotting was performed on whole-cell lysates (WCL) from six NK cell lines using antibodies to phosphotyrosine (Y705)-STAT3 and STAT3. DHL16 cells, which lack STAT3 activation, were used as a negative control. α-Tubulin was used as a control to ensure equal loading of the samples. The names of the cell lines used are indicated above the gel image. The type of the corresponding STAT3 mutation is indicated above the name of the cell lines. (−): No STAT3 mutation; N.D., not determined. ( b ) Representative flow cytometric plots showing the percentage of GFP + cells 3 days (day 0) and 12 days (day 9) post transduction of NKYS cells with EV or STAT3 shRNA after removing IL2 from the culture medium at day 0. ( c ) Quantification of the percentage of GFP + cells post transduction of NKYS cells with EV or STAT3 shRNA at regular time intervals. In one experiment, cells were cultured in the presence of IL2 (5–7 ng ml −1 ) until 3 days (day 0) post transduction and then IL2 was removed from the culture medium. In the second experiment, IL2 was always included post transduction of NKYS cells. Each data point is representative of two biological replicates. ( d ) Representative FACS plots showing the percentage of GFP + cells of YT cell line transduced with EV or STAT3 shRNA 3 days (day 0) or 15 days (day 12) post transduction. ( e ) Quantification of the percentage of GFP + cells by FACS between 3 and 15 days post transduction with EV or STAT3 shRNA. For 1 week before transduction, YT cells were cultured in the presence of IL2. Three days post transduction (day 0), cells were transferred to medium lacking IL2. *: P <0.05, Student’s t -test. ( f ) Representative FACS plots showing the percentage of GFP + cells in EV or STAT3 shRNA transduced KAI3 cells. ( g ) Quantification of the percentage of GFP + cells after transduction of KAI3 cells with EV or STAT3 shRNA. Three days post transduction (day 0), the percentage of GFP + cells was determined by flow cytometry, and cells were switched to NK culture medium with reduced IL2 (25 IU ml −1 ). Data represent means ±s.d. of two biological replicates for panels c , e and g . ( h ) Western blot images of STAT3 knock-down levels are shown for NKYS,YT and KAI3 cell lines on STAT3 shRNA transduced, GFP + sorted cells post transduction with the EV (PLVTH) or STAT3 shRNA (S3S). ( i ) Quantification of the STAT3 protein knock-down levels after normalization to α-Tubulin using the ImageJ program ( http://rsb.info.nih.gov/ij/ ). Full size image Some of the STAT3/STAT5B mutations have been reported in other tumours and are likely oncogenic, but other mutations have not been previously identified. We used several approaches to confirm that these mutations are functionally significant and not passenger mutations or uncommon SNPs. We transduced KAI3 cells, which lack STAT3 or STAT5B mutations, with each of the STAT3 and STAT5B mutants and determined the % of GFP + cells post transduction in regular time intervals. With only two exceptions, all STAT5B- or STAT3-mutant transduced KAI3 cells showed significant progressive positive selection under limiting IL2 concentrations compared with WT transduced cells ( Fig. 3a,b ). STAT3 A702T mutant showed only modest positive selection when compared with WT transduced cells. 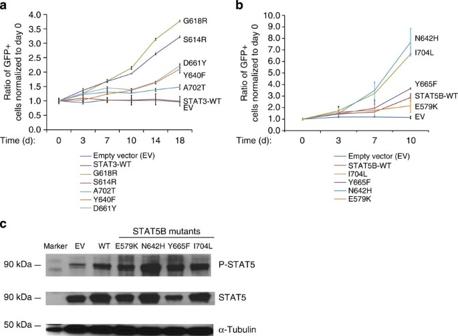Figure 3: Ectopic expression of STAT3 or STAT5B mutants promotes growth in KAI3 cells under limiting IL2 concentrations. (a) Quantification of the percentage of GFP+cells post transduction of KAI3 cells with each STAT3 mutant observed in tumour samples. Transduced cells were cultured in regular IL2 concentrations for 4 days, then switched to limiting (25 IU ml−1) IL2 concentrations. Day 0=4 days post transduction. Each data point shows the means±s.d. of two biological replicates. The average values for the % of GFP+cells at day 0 were 6.9, 3.2, 6.0, 2.8, 4.1, 4.3 and 3.2% for EV, STAT3-WT, S614R, G618R, Y640F, D661Y or A702T transduced cells, respectively. (b) Quantification of the percentage of GFP+cells post transduction of KAI3 cells with each STAT5B mutant observed in tumour samples as ina. Means±s.d. of two independent experiments with replicates are shown (n=4). The average values for the % of GFP+cells at day 0 were 4.8, 6.8, 5.9, 5.7, 8.2 and 6.7% for EV, STAT5B-WT, E579K, N642H, Y665F or I704L-mutant transduced cells, respectively. The percentage of GFP+cells for each sample is normalized to day 0 in botha,b. (c) P-STAT5(Y699) and STAT5 protein expression levels in KAI3 cells transduced with STAT5B mutants are shown by western blot. Six days post transduction, the GFP+population of STAT5B-mutant transduced cells was isolated by FACS, and then placed into culture medium with limiting (25 IU ml−1) concentrations. Whole-cell lysates were collected 11 days post transduction. One experiment representative of three experiments is shown. Figure 3: Ectopic expression of STAT3 or STAT5B mutants promotes growth in KAI3 cells under limiting IL2 concentrations. ( a ) Quantification of the percentage of GFP + cells post transduction of KAI3 cells with each STAT3 mutant observed in tumour samples. Transduced cells were cultured in regular IL2 concentrations for 4 days, then switched to limiting (25 IU ml −1 ) IL2 concentrations. Day 0=4 days post transduction. Each data point shows the means±s.d. of two biological replicates. The average values for the % of GFP + cells at day 0 were 6.9, 3.2, 6.0, 2.8, 4.1, 4.3 and 3.2% for EV, STAT3-WT, S614R, G618R, Y640F, D661Y or A702T transduced cells, respectively. ( b ) Quantification of the percentage of GFP + cells post transduction of KAI3 cells with each STAT5B mutant observed in tumour samples as in a . Means±s.d. of two independent experiments with replicates are shown ( n =4). The average values for the % of GFP + cells at day 0 were 4.8, 6.8, 5.9, 5.7, 8.2 and 6.7% for EV, STAT5B-WT, E579K, N642H, Y665F or I704L-mutant transduced cells, respectively. The percentage of GFP + cells for each sample is normalized to day 0 in both a , b . ( c ) P-STAT5(Y699) and STAT5 protein expression levels in KAI3 cells transduced with STAT5B mutants are shown by western blot. Six days post transduction, the GFP + population of STAT5B-mutant transduced cells was isolated by FACS, and then placed into culture medium with limiting (25 IU ml −1 ) concentrations. Whole-cell lysates were collected 11 days post transduction. One experiment representative of three experiments is shown. Full size image Western blot analysis in cell lines clearly demonstrated an association of STAT3 mutations with increased phosphorylation. As there are no cell lines with STAT5B mutations, we measured the phosphorylation of STAT5B proteins in STAT5B-mutant transduced KAI3 cells and found it to be clearly increased compared with WT transduced cells ( Fig. 3c ). Next, we transduced STAT5B mutants (N642H and I704L) into primary human NK cells obtained through coculture with engineered K562 cells, K562-Cl9-mb21, and observed robust promotion of cell growth in mutant compared with WT transduced cells ( Fig. 4 ). Intriguingly, the effect of STAT5B N642H was prominent and the strongest among all mutants tested in KAI3 cells or normal NK cells. 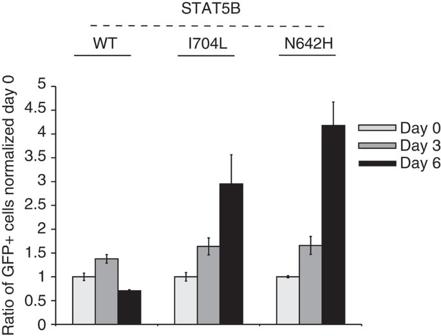Figure 4: Ectopic expression of STAT5B I704L or N642H mutants promotes growth of primary human NK cells. Quantification of the percentage of GFP+cells post transduction of primary NK cells with STAT5B-WT or each of two STAT5B mutants (I704L or N642H) at 3-day intervals. The percentage of GFP+cells for each sample is normalized to day 0. Day 0 indicates 5 days post transduction. The average % of GFP+cells at day 0 was 4.6, 4.9 and 4.8% for STAT5B-WT, N642H or I704L transduced cells, respectively. Data are mean±s.d. of two biological replicates. Dead cells were stained with 0.5 μM of DAPI (Biolegend, cat. no: 422801) to exclude them from quantification. Figure 4: Ectopic expression of STAT5B I704L or N642H mutants promotes growth of primary human NK cells. Quantification of the percentage of GFP + cells post transduction of primary NK cells with STAT5B-WT or each of two STAT5B mutants (I704L or N642H) at 3-day intervals. The percentage of GFP + cells for each sample is normalized to day 0. Day 0 indicates 5 days post transduction. The average % of GFP + cells at day 0 was 4.6, 4.9 and 4.8% for STAT5B-WT, N642H or I704L transduced cells, respectively. Data are mean±s.d. of two biological replicates. Dead cells were stained with 0.5 μM of DAPI (Biolegend, cat. no: 422801) to exclude them from quantification. Full size image Next, we evaluated the expression of known STAT5B targets, IL2R α (ref. 12 ), BCL-XL [13] , BCL2 (ref. 14 ), MIR155HG (ref. 15 ) and HIF2 α (ref. 16 ) in KAI3 cells transduced with STAT5B mutants (N642H and I704L) and observed significantly higher expression compared with WT or EV transduced cells ( Fig. 5a–e ), indicating that the mutants are functionally active and upregulate oncogenic STAT5B targets, which in part accounts for better promotion of growth in NK cells. Next, we performed ChIP-q-PCR on STAT5 binding sites for these genes. Compared with KAI3 cells transduced with EV or WT STAT5B, a robust increase in occupancy of STAT5 binding sites were observed in STAT5B-N642H transduced KAI3 cells ( Fig. 5f–j ), indicating that increased STAT5B binding due to the mutation upregulates the expression of the target genes. Altogether, these results suggest that the STAT3/STAT5B mutations are oncogenic, driver mutations. 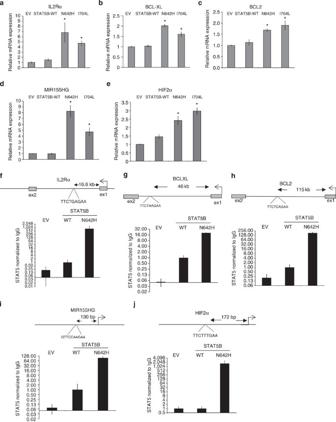Figure 5: STAT5B target genes are transcriptionally upregulated in STAT5B-mutant transduced cells through direct binding to conserved STAT5 binding sites. Relative mRNA expression ofIL2Rα (a),BCL-XL(b),BCL2(c),MIR155HG(d) and,HIF2α (e) is shown in control vector or STAT5B-mut transduced cells obtained by sorting GFP+cells 10 days post transduction, and then culturing for 5 days and 2 days in culture medium with regular or limiting (25IUml−1) IL2 concentrations, respectively. Means±s.d. of two independent experiments (total combined samples=4) are shown. *P<0.01 compared with WT, Student’st-test. ChIP-q-PCR results for known STAT5 binding sites are shown forIL2Rα (f),BCL-XL(g),BCL2(h),MIR155HG(i) andHIF2α (j) in EV, STAT5B-WT or STAT5B-N642H transduced KAI3 cells. Data are mean±s.d. of four replicates. STAT5 pull-down normalized to IgG control as a fold difference compared with STAT5B-WT sample is shown in the y-axis using a log scale. STAT5B consensus sites and their approximate distance to the TSS sites are indicated. Figure 5: STAT5B target genes are transcriptionally upregulated in STAT5B-mutant transduced cells through direct binding to conserved STAT5 binding sites. Relative mRNA expression of IL2R α ( a ), BCL-XL ( b ), BCL2 ( c ), MIR155HG ( d ) and, HIF2 α ( e ) is shown in control vector or STAT5B-mut transduced cells obtained by sorting GFP + cells 10 days post transduction, and then culturing for 5 days and 2 days in culture medium with regular or limiting (25IUml −1 ) IL2 concentrations, respectively. Means±s.d. of two independent experiments (total combined samples=4) are shown. * P <0.01 compared with WT, Student’s t -test. ChIP-q-PCR results for known STAT5 binding sites are shown for IL2R α ( f ), BCL-XL ( g ), BCL2 ( h ), MIR155HG ( i ) and HIF2 α ( j ) in EV, STAT5B-WT or STAT5B-N642H transduced KAI3 cells. Data are mean±s.d. of four replicates. STAT5 pull-down normalized to IgG control as a fold difference compared with STAT5B-WT sample is shown in the y-axis using a log scale. STAT5B consensus sites and their approximate distance to the TSS sites are indicated. Full size image STAT5B N642H is the most frequent mutation identified in γδ-PTCLs and appears to have the highest functional potency. Hence, we sought to determine the molecular basis of the functional alterations resulting from this mutation through structural analysis. To mimic homodimerization, we docked a tyrosine-phosphorylated STAT5B peptide into the WT and mutant SH2 domains ( Fig. 6a–c ). Molecular docking showed that the peptide has a significantly higher binding affinity to the N642H mutant than the WT ( Fig. 6d ) largely due to the direct electrostatic interaction of the mutant histidine with the phosphotyrosine. To confirm these modelling studies, we produced non-phosphorylated WT and N642H STAT5B (residues 128 to 717), purified each to homogeneity, and performed SPR studies. The WT and mutant STAT5B proteins were coupled to individual channels of a CM5 SPR chip, and the phosphopeptide KAVDG(p)YVKPQI was passed over each channel at increasing concentrations (0.8 to 100 μM) in duplicates. The binding affinity of the peptide to the WT and N642H mutant was determined by fitting the equilibrium saturation point as a function of peptide concentration. The dissociation constants for the N642H mutant and WT STAT5B on average were 3.2 and 15.6 μM, respectively ( Fig. 6e ). While these measurements represent a ~fivefold difference for the peptide to the monomeric STAT5B-WT compared with N642H mutant, it is important to note that phosphoSTAT5B forms a homodimer and thus there are two phosphotyrosine binding sites. Consequently, K Dimer = K Monomer1 · K Monomer2 that translates to a 25-fold increased association constant for the dimer. Hence, the homodimeric N642H mutant is substantially more stable than the WT. This finding supports the molecular model and the in vitro cell based assay observations. 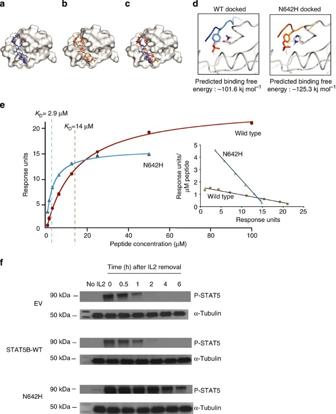Figure 6: Three-dimensional modelling and SPR analysis of the N642H mutant shows stronger affinity for the phosphorylated tyrosine Y699. The phosphorylated STAT5B peptide involved in homodimerization was docked into the SH2 domain of either WT (a) or N642H (b) STAT5B. The overlay of these structures (c) shows little difference in the docking poses. In both cases, the N642 or H642 residue was found to be in close proximity to the phosphorylated tyrosine on the STAT5B peptide (d). The binding energy of these docked structures was calculated for both the WT (−101.5 kJ mol−1) and N642H (−125.3 kJ mol−1). (e) SPR binding isotherms of phosphopeptide with STAT5B-WT (brown circles) and N642 mutant (blue triangles) of a representative experiment is shown. CalculatedKDvalues of 14 and 2.9 μM for STAT5B-WT and N642H mutant, respectively, are indicated by vertical lines for the representative experiment. An inset shows the Scatchard plot of the same data. The experiment was repeated for four times, and the means±s.d. ofKDvalues for WT and N642H are 15.6±1.4 μM and 3.23±0.33 μM, respectively.P<0.01 for N642H compared with WT, Student’st-test. (f) Western blot image showing P-STAT5(Y699) and STAT5 levels before or after culturing EV, STAT5B-WT or N642H mutant transduced, GFP-sorted YT cells in the absence (no IL2) or the presence of IL2. YT cells were cultured in the absence of IL2 in each stage of the experiment including 1 week before transduction. The image is representative of two independent western blots. Figure 6: Three-dimensional modelling and SPR analysis of the N642H mutant shows stronger affinity for the phosphorylated tyrosine Y699. The phosphorylated STAT5B peptide involved in homodimerization was docked into the SH2 domain of either WT ( a ) or N642H ( b ) STAT5B. The overlay of these structures ( c ) shows little difference in the docking poses. In both cases, the N642 or H642 residue was found to be in close proximity to the phosphorylated tyrosine on the STAT5B peptide ( d ). The binding energy of these docked structures was calculated for both the WT (−101.5 kJ mol −1 ) and N642H (−125.3 kJ mol −1 ). ( e ) SPR binding isotherms of phosphopeptide with STAT5B-WT (brown circles) and N642 mutant (blue triangles) of a representative experiment is shown. Calculated K D values of 14 and 2.9 μM for STAT5B-WT and N642H mutant, respectively, are indicated by vertical lines for the representative experiment. An inset shows the Scatchard plot of the same data. The experiment was repeated for four times, and the means±s.d. of K D values for WT and N642H are 15.6±1.4 μM and 3.23±0.33 μM, respectively. P <0.01 for N642H compared with WT, Student’s t -test. ( f ) Western blot image showing P-STAT5(Y699) and STAT5 levels before or after culturing EV, STAT5B-WT or N642H mutant transduced, GFP-sorted YT cells in the absence (no IL2) or the presence of IL2. YT cells were cultured in the absence of IL2 in each stage of the experiment including 1 week before transduction. The image is representative of two independent western blots. Full size image To address whether the STAT5B-N642H mutation is associated with prolonged STAT5B activation in the presence of acute JAK-STAT5 pathway activation, we performed western blot on IL2-activated YT cells in a time-course experiment to evaluate P-STAT5 expression. The JAK-STAT5 pathway is known to be inducible in this cell line [17] . We incubated EV, STAT5B-WT or N642H-mutant transduced YT cells with IL2 for 30 min, and evaluated P-STAT5 expression up to 6 h after IL2 withdrawal. P-STAT5 expression disappeared 1 h after transient IL2 stimulation in EV or STAT5B-WT transduced cells whereas it persisted for >6 h in N642H transduced cells ( Fig. 6f ). These results suggest that the N642H mutation increases affinity of phospho-STAT5B dimerization and thereby resulting in far more persistent activation. We next tested whether a JAK1/2 inhibitor can inhibit cell growth of STAT5B or STAT3-mutant transduced KAI3 cells. Most NKCL and γδ-PTCL cell lines are still dependent on IL2 which signals mainly through JAK1/2 to activate STAT3 and STAT5 (refs 18 , 19 ). JAK inhibitors are expected to be effective in interrupting this signalling pathway in cells with WT STAT3 and STAT5. However, it is unclear whether the inhibitor would effectively inhibit this pathway at a tolerable dosage in cells harbouring the mutants. We treated STAT3 or STAT5B mutant and WT transduced KAI3 cells with 0.5 μM AZD1480, a selective JAK1/2 inhibitor [20] . We quantified viable cells at 72 h post treatment and observed inhibition of growth in all the mutant STAT3 and STAT5B transduced cells ( Fig. 7a,b ). With higher concentrations of AZD1480, we observed up to 60% inhibition in STAT5B N642H-mutant transduced cells ( Fig. 7c , right), associated with reduced STAT5 phosphorylation in a dose-dependent manner ( Fig. 7d ). Next, we treated YT and NKYS cells, which have STAT3 mutations, with the JAK1/2 inhibitor and observed dose-dependent inhibition of cell growth ( Fig. 7e ). These data suggest that JAK1/2 inhibitors may have therapeutic efficacy for NKTCL and γδ-PTCL patients with the mutations. This may have immediate clinical implication as JAK1/2 inhibitors are already approved for myeloproliferative disorders [21] , [22] so they are available for trials in NKTCL or γδ-PTCL patients while STAT3 and STAT5B inhibitors are still not clinically available. Further development of small-molecule inhibitors targeting STAT3 or STAT5B dimerization or DNA binding may synergize with JAK1/2 inhibitors to improve the outcome in these diseases with currently dismal prognosis. 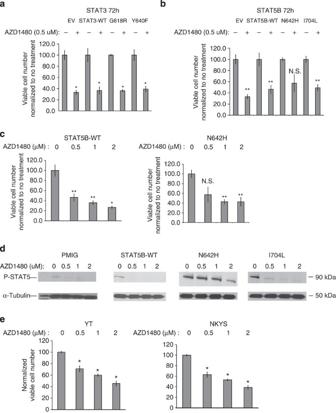Figure 7: AZD1480 inhibits STAT3/STAT5B-mutant transduced NK cells. STAT3-mutant (a) or STAT5B mutant (b) transduced, GFP+-sorted KAI3 cells were treated with 0.5 μM AZD1480 for 72 h. Viable cell number was determined using Vi-cell XR cell viability analyser (Beckman Coulter Inc.) as described in Supplementary Methods and normalized to the corresponding untreated sample. Means±s.d. of two biological replicates are shown. (c) Normalized viable cell number of STAT5B-WT (left) or N642H-mutant (right) transduced KAI3 cells treated with progressively increasing doses of AZD1480 for 72 h. Each column represents mean±s.d. of three biological replicates. (d) P-STAT5 (Y699) levels were analysed by western blot on EV, STAT5B-WT, N642H or I704L transduced KAI3 cells treated with progressively increasing doses (0.5 μM, 1 or 2 μM) of AZD1480 for 4 h (e) Normalized numbers of viable STAT3-mutated NKYS and YT cells treated as in (c) are shown *P<0.01 versus no treatment; **P<0.05 versus no treatment; Student’st-test. NS: not significant. Figure 7: AZD1480 inhibits STAT3/STAT5B-mutant transduced NK cells. STAT3-mutant ( a ) or STAT5B mutant ( b ) transduced, GFP + -sorted KAI3 cells were treated with 0.5 μM AZD1480 for 72 h. Viable cell number was determined using Vi-cell XR cell viability analyser (Beckman Coulter Inc.) as described in Supplementary Methods and normalized to the corresponding untreated sample. Means±s.d. of two biological replicates are shown. ( c ) Normalized viable cell number of STAT5B-WT (left) or N642H-mutant (right) transduced KAI3 cells treated with progressively increasing doses of AZD1480 for 72 h. Each column represents mean±s.d. of three biological replicates. ( d ) P-STAT5 (Y699) levels were analysed by western blot on EV, STAT5B-WT, N642H or I704L transduced KAI3 cells treated with progressively increasing doses (0.5 μM, 1 or 2 μM) of AZD1480 for 4 h ( e ) Normalized numbers of viable STAT3-mutated NKYS and YT cells treated as in ( c ) are shown * P <0.01 versus no treatment; ** P <0.05 versus no treatment; Student’s t -test. NS: not significant. Full size image Although STAT3 or STAT5B mutations have been reported in malignancies such as B-cell lymphomas [23] , angioimmunoblastic T-cell lymphoma [24] , CD30 + T-cell lymphoma [25] , the indolent LGLL diseases [26] , [27] , [28] and recently in T-cell prolymphocytic leukaemia [29] , which also included functional characterization of STAT5 mutations, our study describes prevalent activating STAT5B and STAT3 mutations in aggressive lymphomas of NK and γδ-T cell of origin. Importantly, we provided strong in vitro functional data that support an oncogenic role of these mutants as well as mechanistic insight into how the N642H mutant acquires enhanced functional activities. The frequency of activating STAT3 mutations was much higher in NK (50%) and γδ-T cell lines (67%) compared with NKTCL (5.9%) or γδ-PTCL patient samples (8.3%). This suggests that JAK-STAT3 pathway activation may be more critical in cell survival independent of stromal components and that consequently the activating mutations are selectively enriched in cell lines. Intriguingly, STAT5B mutations were far more frequent in γδ-T-cell lymphomas including multiple subtypes: HS, EATL type II and other mucocutaneous γδ-PTCL (34.9%) than in NKTCL cases (5.9%) suggesting a pivotal role of STAT5B in γδ-PTCL pathogenesis. Patient samples and cell lines The phenotypic characteristics of all NKTCL, δγ-PTCL and EATL type II cases ( n =94), NK and δγ-T cell lines ( n =9) used in this study are summarized in Supplementary Table 2 . Informed consent was obtained from all patients in accordance with the Declaration of Helsinki, and use of patient materials and information was approved by the institutional review boards of the UNMC, West China Hospital Sichuan University, and the participating institutions of the Tenomic Consortium. KHYG1, KAI3 cell lines were obtained from the Health Science Research Resource (Osaka, Japan). YT and NK-92 cell lines were provided by the German Collection of Microorganism and Cell Culture (GCMCC) (DSMZ, Braunschweig, Germany). Two NK cell lines (SNK6, NKYS) and the γδ-T cell lines (SNT8, SNT13, and SNT15) were obtained from Dr Norio Shimizu (Tokyo Medical and Dental University). Culture conditions of NK and γδ-T cell lines were as described previously [30] , [31] . The DHL16 cell line, purchased from ATCC (American Type Culture Condition), was cultured in RPMI-1640 (Gibco-Invitrogen) including 10% FBS; penicillin G (100 units ml −1 ) and streptomycin (100 μg ml −1 ) at 37 °C in 5% CO 2 . WTS and data analysis RNA sequencing was performed on resting NK cells, NK cells activated by IL2 or by K562-Clone9-mb21, 17 NKTCL cases and 3 NK cell lines. Briefly, 100-bp paired-end libraries were prepared with the TrueSeq RNA preparation kit (Illumina Inc., San Diego, CA), and high-throughput sequencing was performed at the UNMC Next Generation Sequencing Core facility and Tufts University (TUCF) Genomics Core Facility using Illumina Genome Analyzer IIX or HiSeq 2000 Sequencing systems. FASTQC reports were evaluated for each sample to evaluate the quality of basic statistics. Two different pipelines were used to generate the SNVs. The main pipeline used for SNV detection was described previously [32] with the following addition. In addition to the NCBI SNP database (dbSNP) and 1,000 Genomes project [33] , three normal NK samples were used to filter out the SNPs. The presence of the SNVs was evaluated by visualizing the SNVs using Integrative Genomics Viewer software (IGV) ( http://www.broadinstitute.org/igv ). Finally, the Cosmic release v69 ( http://cancer.sanger.ac.uk/cancergenome/projects/cosmic/ ) was used to annotate the variants observed in previous studies. The secondary pipeline used for SNV detection is as follows: The reads were aligned to the human reference genome (NCBI GRCh37) using the BWA aligner [34] with paired-end (sampe) mode and with default options. After merging BAM files, PCR duplications were also removed. Then, GATK tool [35] was used to realign indel-containing reads to the reference genome. After realignment, GATK UnifiedGenotyper was used to generate SNP and indel callsets for 24 (21 malignant and three normal NK samples) RNA-Seq samples, using a merged BAM file including all 24 data sets with specific IDs. Variant Quality Score Recalibration filter was applied using the GATK resource bundle 1.2 to help minimize false positives. Then, ANNOVAR tool [36] , version 2013-02-11, was used to annotate the detected SNPs and indels. For gene and filter annotation, the April 2012 version of the annotation database (hg191000g2012apr) and dbSNP version 137 was used. For comparison against the 1,000 Genomes Project, the data 1000g2012apr was used. Lastly, the SNVs present in three normal NK samples were filtered out. The basic statistics of RNA-Seq are shown in Supplementary Table 3 . Furthermore, the number of SNVs and their annotations identified by the primary RNA-Seq pipeline for 17 NKTCL cases are shown in Supplementary Fig. 3 and Supplementary Table 4 , respectively. Whole genome amplification Whole genome amplification (WGA) of the NKTCL ( n =20) or γδ-PTCL ( n =4) cases and KAI3 cell line was performed using the Repli-g kit (Qiagen Inc., Valencia, CA). 50 ng of tissue material was used as a template for amplification. The sensitivity of mutation detection was evaluated by applying Sanger sequencing on the G to A mutation detected in the intron4/exon5 splice junction of PRDM1 detected previously ( Supplementary Fig. 4A ) [30] . Uniform linear amplification of genomic DNA from each NK sample was tested with PCR, which generated~3 kb amplicons using KAI3 cell line or NKTCL cases ( Supplementary Fig. 4B,C ). In addition, WGA DNA from NKTCL cases was run on TAE-agarose gels, which showed that WGA DNA contains large fragments (>10 kb) ( Supplementary Fig. 4D ). Mutation validation by Sanger sequencing Sanger sequencing was performed on DNA from cryopreserved or FFPE tissues, or cDNA if only RNA was available. Sequencing was focused on the SH2 domain of STAT3 and STAT5B and the previously reported mutation hotspots for JAK3 . The genomic DNA sequences around the JAK3 A572V, A573V and V722I SNVs was obtained using UCSC ( http://genome.ucsc.edu/ ) genome browser. PCR primers covering SNVs were designed with the PrimerQuest software (IDT DNA technologies, Coralville, IA). The primers were optimized with gradient PCR, and the forward and reverse primers used for PCR amplification of WGA or FFPE gDNA or cDNA samples were used for Sanger sequencing. Analysis of the sequences was performed using Vector NTI 10.3.0 (Invitrogen, Carlsbad, CA) and Sequence Scanner Software v1.0 (Applied Biosystems Inc.).The primers used for Sanger sequencing are shown in Supplementary Table 5 . NK cell isolation and activation for RNA-Seq Primary human NK cells were isolated from peripheral blood lymphocytes using a human NK cell isolation kit (Miltenyi Biotec, Auburn, CA) as described previously [37] . The purity of NK cells was evaluated by CD56-APC and CD3-PE double staining, and samples with >95% CD56 + CD3 − cells were used for RNA-Seq. Resting NK cells were cultured in the presence of 100 IU of IL2 for 48 h to obtain activated NK cells. Higher levels of NK cell activation were achieved by coculturing freshly isolated peripheral blood lymphocytes with engineered K562 cells, K562-Clone9-mb21, as described in detail before [37] , [38] . Quantitative reverse transcription PCR (q-RT–PCR) mRNA expression was determined with q-RT–PCR. RNA isolation and reverse transcription were performed as described previously [37] , [39] . Real-time PCR was performed using DyNAmo HS SYBR Green qPCR Kit (Thermo Scientific Inc.) with CFX Connect (Bio-Rad, Hercules, CA) real-time thermocycler. Melting curve analysis was performed to ensure amplification specificity. The ΔΔCt method was used to calculate the relative mRNA expression level. RPL13A was used for normalization of gene expression. Q-RT–PCR primers used in this study are as follows: BCL-XL forward: 5′- CTTACCTGAATGACCACCTAGAG -3′; BCL-XL reverse: 5′- AGGAACCAGCGGTTGAAG -3′; IL2R α forward: 5′- AGCGAGCGCTACCCACTTCTAAAT -3′; IL2R α reverse: 5′- AGGGTGGAGAGAGTTCCATACCAT -3′; BCL2 forward: 5′- CATGTGTGTGGAGAGCGT CAA -3′; BCL2 reverse: 5′- CAGAGACAGCCAGGAGAAATCA -3. MIR155HG forward: 5′- ACGGTTGTGCGAGCAGAGAATCTA -3′; MIR155HG reverse: 5′- CTCATCTAAGCCTCACAACAACCT -3′; HIF2 α forward: 5′- GTGCTCCCACGGCCTGTA -3′; HIF2 α reverse: 5′- TTGTCACACCTATGGCATATCACA -3′. Western blot Western blot was performed as described previously with the following modifications [30] . RIPA buffer supplemented with a protease inhibitor cocktail (Sigma-Aldrich, St Louis, MO) and phosphatase inhibitor cocktails 2 and 3 (Sigma-Aldrich) was used to prepare the whole-cell lysate. Twenty micrograms protein/sample was used for western blot. BSA (Sigma-Aldrich) was used instead of non-fat dry milk during blocking. The primary antibodies used for western blotting are as follows: STAT3 (Cell Signaling Inc., Danvers, MA), STAT5 (3H7) Rabbit mAb #9358 (Cell Signaling), phospho-STAT5 D47E7 Rabbit mAb # 4322 (Cell Signaling), phospho-STAT3 (Cell Signaling) and α-Tubulin (Sigma-Aldrich). The working dilution of α-Tubulin is 1:50,000. The working dilution for all other antibodies is 1:1,000. Uncropped representative WB images are shown in Supplementary Fig. 5 . STAT3 shRNA expression in NK cell lines The lentiviral construct used for STAT3 knock-down was described previously [40] . Lentiviral transduction of NK cell lines or DHL16 was performed following the protocol used for retroviral transduction [37] with the following modifications: 4 μg PLVTH or PLVTH-S3S was cotransfected with 2 μg of PMD2G and 2 μg psPAX2 packaging constructs into the 293T cell line to generate lentiviral particles. Transduction was performed once rather than twice. Transduction efficiency was determined with fluorescence-activated cell sorting (FACS) 3 days post transduction. Generation and expression of the STAT3 or STAT5B constructs WT STAT5B was PCR cloned with the high-fidelity PfuUltra II Fusion HS DNA Polymerase (Agilent Technologies, Palo Alto, CA) using NK92 cell line cDNA as the template and then cloned into the multiple cloning site of the pMIG expression vector using NotI and SalI restriction sites. Similarly, WT STAT3 was PCR cloned into pMIG from KAI3 cell line cDNA using NotI and SalI sites. Diagnostic mapping and full insert sequencing was performed. These WT STAT3 or STAT5B constructs were used as templates for site-directed mutagenesis to generate the STAT3 or STAT5B mutants used for functional studies as described below apart from the STAT3-Y640F-pMIG construct, which was PCR cloned with PfuUltra II Fusion HS DNA Polymerase using the cDNA from NKYS cells, which have the STAT3 Y640F mutation. STAT3 or STAT5B SNVs observed in NKTCL, γδ-PTCL or EATL type II samples (patient samples or cell lines) were generated using the Quick-Change Site-Directed Mutagenesis Kit (Agilent technologies, Santa Clara, CA) according to the manufacturer’s instructions using WT STAT3 or STAT5B-pMIG vectors ( Supplementary Fig. 6 ). Diagnostic restriction mapping and full sequencing of the inserts were performed to ensure the presence of introduced mutation and absence of another SNV. The primers used for site-directed mutagenesis (SDM) are as follows: STAT3-S614R-SDM-F: 5′- GAAAGCAGCAAAGAAGGACGCGTCACTTTCACTTGG -3′; STAT3-S614R-SDM-R: 5′- GTGACGCCTCCTTCTTTGCGGCTTTCACTGAATCTT -3′; STAT3-G618R-SDM-F: 5′- GAAAGCAGCAAAGAAGGACGCGTCACTTTCACTTGG -3′; STAT3-G618R-SDM-R: 5′- CCAAGTGAAAGTGACGCGTCCTTCTTTGCTGCTTTC -3′; STAT3- D661Y-SDM-F: 5′- TGGGCTATAAGATCATGTATGCTACCAATATCCTGG -3′; STAT3-D661Y-SDM-R: 5′- CCAGGATATTGGTAGCATACATGATCTTATAGCCCA -3′; STAT3-A702T-SDM-F: 5′- AGCTGACCCAGGTAGCACTGCCCCATACCTGAAG -3′; STAT3- A702T-SDM-R: 5′- CTTCAGGTATGGGGCAGTGCTACCTGGGTCAGCT -3′; STAT5B-E579K-SDM-F: 5′- GGTTTGACGGTGTGATGAAAGTGTTAAAAAAACATC -3′; STAT5B-E579K-SDM-R: 5′- GATGTTTTTTTAACACTTTCATCACACCGTCAAACC -3′; STAT5B-N642H-SDM-F: 5′- GGAAAGAATGTTTTGGCATCTGATGCCTTTTACC -3′; STAT5B-N642H-SDM-R: 5′- GGTAAAAGGCATCAGATGCCAAAACATTCTTTCC -3′; STAT5B-Y665F-SDM-F: 5′- GCTTGGGAGACTTGAATTTCCTTATCTACGTGTTTC -3′; STAT5B-Y665F-SDM-R: 5′- GAAACACGTAGATAAGGAAATTCAAGTCTCCCAAGC -3′; STAT5B-I704L-SDM-F: 5′- GGATACGTGAAGCCACAGCTCAAGCAAGTGGTCCCTG -3′; STAT5B-I704L-SDM-R: 5′- CAGGGACCACTTGCTTGAGCTGTGGCTTCACGTATCC -3′. Retroviral transduction of NK cell lines was performed as previously described [39] with the following modifications: 4 μg of pMIG or pMIG vectors expressing WT or mutated STAT3/STAT5B gene was cotransfected with 4 μg of the packaging construct PCL-Ampho into the 293T cell line. A single transduction was performed. Transduction efficiency was determined with flow cytometry on GFP + cells 2–4 days post transduction. KAI3 cells were cultured in the presence of 20% FBS to increase transduction efficiency. Conditioning primary NK cells for retroviral transduction Primary human NK cells were expanded using a special ex vivo system that involves coculturing primary human NK cells with an engineered NK cell target, K562-Cl9-mb21, which activates and induces proliferation of NK cells robustly as described before [37] , [39] . The expansion procedure is described briefly as follows: First, primary human NK cells were isolated by negative selection using EasySepHuman NK cell enrichment kit (Stemcell technologies,Vancouver,Canada). Then, primary NK cells were admixed in a 1:2 ratio with 100 Gr irradiated K562-Cl9-mb21cells, which express CD86, 4-1BBL and mIL21 on their surface, and cultured in NK cell expansion medium [38] . Cells were spun down at 400 g for 5 min, and the culture medium was renewed every 3 days with fresh culture medium, keeping the cell density at 250,000 cells per ml after every subculture. Nine days after coculture started, cells were immunostained with CD56-PE (Biolegend, San Diego, CA) and CD3-FITC (Biolegend) antibodies to determine the NK cell purity by FACS. On the same day purity was determined, primary NK cells were transduced with WT or mutant STAT5B retroviral constructs. Determination of positive/negative selection of transduced cells STAT3 shRNA or STAT3/STAT5B mutant transduced NK cell lines were tracked by quantification of the GFP + cells using flow cytometry after transduction to determine negative or positive selection of cells, respectively, because GFP was used as the marker of transduction. The following flow cytometers were used for determination of GFP + cells: FACS Calibure (BD Biosciences), BD LSRFortessa (BD Biosciences) and Gallious (Beckman Coulter Inc.) Autofluorescent cells, which emit both green and orange, represent false positive, untransduced cells, were filtered out through proper gating. During quantification of GFP + cells in transduced primary NK cells, dead cells were labelled and filtered out by staining the cells with 0.5 ug ml −1 DAPI (Biolegend, cat.no: 422801) for 10 min before flow cytometry. ChIP-q-PCR Ten million cells isolated from GFP-sorted, EV, STAT5B-WT or N642H-mutant transduced KAI3 cells were used for chromatin immunoprecipitation using ChIP-IT Express Enzymatic (Active Motif, Carlsbad, CA) following the manufacturer’s recommendations.The procedure is described briefly as follows: the enzymatic digestion time was optimized as 10 min based on the TAE-agarose gel image. Cells (10*10 6 ) per sample were fixed with 1% formaldehyde. After enzymatic fragmentation, STAT5 (3H7) Rabbit mAb #9358 (Cell Signaling Inc.) and rabbit anti-IgG Control (Abcam Inc., Cambridge, MA) antibodies were used side-by-side for immunoprecipitations. Twenty micrograms of chromatin/reaction was immunoprecipitated using dilutions of STAT5 or IgG antibody based on manufacturers’ recommendations. After elution of DNA, reversal of DNA cross-links, and proteinase K treatment, q-PCR was performed using 2 μl of gDNA in replicate. STAT5 immunoprecipated DNA levels were normalized to the levels of IgG immunoprecipitated DNA for each sample. STAT5 binding sites reported before for IL2Ra (ref. 12 ), BCL2 (ref. 14 ), BCL-XL (ref. 12 ), HIF2 α (ref. 16 ) and MIR155HG (ref. 15 ) were evaluated. The sequences of ChIP-q-PCR primers used in this study is as follows: IL2R α-ChIP-q-PCR-F: 5′- AAAACCAATTTCTTGGGATGG -3′; IL2Rα -ChIP-q-PCR-R: 5′: AGGGGAAATTCCGTTGAGTT -3′; BCL2 ChIP-q-PCR-F: 5′- ACTTTACATTTCTGTTGTGTTTACAGC -3′, BCL2 ChIP-q-PCR-R: 5′- ATTCATACATATGCACACGCACA -3′; BCL-XL ChIP-q-PCR F: 5′- AATTCAGCTGCCAGCCTCT -3′, BCL-XL ChIP-q-PCR R: 5′- CAACCGCTTCCTTTTCTGAG -3′, HIF2α (EPAS1) ChIP-q-PCR F: 5′- CAGTGTCCTGAGACTGTATG -3′, HIF2α (EPAS1) ChIP-q-PCR R: 5′- CTGTCAGACCCGAAAAGA -3′, MIR155HG ChIP-q-PCR F: 5′-GAAAGGGAAAGGGGAAAACA-3′, MIR155HG ChIP-q-PCR R: 5′-CGAACGTGCGACCCTTTTAT-3′. AZD1480 treatment of mutant STAT3- or STAT5B-transduced KAI3 cells In all, 25,000 KAI3 cells were seeded in 2 ml inside 24-well plates in replicates or triplicates and treated with 0, 0.5, 1 or 2 μM of AZD1480 for 72 h. Seventy-two hours post treatment, the total viable cell number in each well was quantified using a Vi-cell XR Cell Viability Analyzer (Beckman Coulter Inc.) according to the manufacturer’s instructions. Total cell number in each treated sample was normalized to that of the untreated control cells. Three-dimensional structural modelling of the STAT5B-N642H mutant The STAT5B structure was modelled on the available STAT5A structure (PDB ID: 1Y1U) using the program MODELLER [41] . There was little difference in the SH2 domains as these two proteins have extremely similar primary sequences. Then, the modelled STAT5B SH2 domain was compared with other proteins containing SH2 domains that had been cocrystallized with peptides (v-SRC, GRB2, SH2B, NCK2) which showed the site of the N642H was directly located in the key binding pocket of the phosphorylated tyrosine. Phosphorylated self-peptide (STAT5B: VDG-PTR-VKPQ) was docked into the SH2 domain of WT-STAT5B or N642H STAT5B, respectively. Protein–protein docking was done with the FFT-based docking tool ClusPro [42] on a dedicated server. Key binding residues (STAT5B: R618, S620, N621, K600, N642) were specified based on previous peptide–SH2 domains cocrystallized structures (PDB ID: 2HDX, 1SHA, 2CIA, 1TZE). The best docking results were selected based on an electrostatically favoured scoring function. ClusPro docking server first clustered 1,000 ligand positions with the lowest energy score according to the 9 angstrom C-alpha RMSD radius and then ranked the best model. With the energy-minimized protein-peptide docked model, the binding energy of the complex was calculated with MolDock [43] . Surface plasmon resonance binding assay For surface plasmon resonance, WT and N642H-mutant STAT5B (residues between 128aa-717aa, NM_012448) was PCR cloned into the SMT3-pET28b+ plasmid using the BamHI and XhoI cloning sites. BclI instead of BamHI restriction site was used in the forward primer to prevent digestion of STAT5B due to the presence of an internal BamHI site. A TGA stop codon was included in the reverse primer so that C-term His was not expressed. High-fidelity PfuUltra II Fusion HS DNA Polymerase (Agilent Technologies, Palo Alto, CA) was used to amplify STAT5B insert from STAT5B-WT-pMIG vector. Diagnostic mapping and Sanger sequencing of the inserts and the integration sites were performed to check the quality of the clones. WT and mutant STAT5B expression was performed as follows: Plasmid DNA was transformed into BL21 (DE3) Codon Plus RIL competent cells (Agilent Technologies) and plated on LB agar plates with chloramphenicol (Cam) and kanamycin (Kan). Single colonies were selected and grown in LB media with Cam and Kan overnight at 37 °C. Overnight culture of 6 × 6 ml was used to inoculate 6 × 1 l LB media with Kan and Cam. Cultures were grown at 37 °C to an optical density of 0.6, then flasks were moved to a precooled shaker at 18 °C. Cultures were grown at 18 °C until they reached an optical density between 0.9and 1.1. Protein expression was induced with a final concentration of 500 μM isopropyl-β- D -thiogalactoside, and cells were allowed to grow 16–20 h at 18 °C with continued shaking. Cells were harvested by centrifugation, resuspended in PBS and frozen at −20 °C until purification. His6-SMT fusions of both WT and N642 mutant STAT5B were purified as previously published [44] . Briefly, cells were thawed and lysed by French pressure cell with DNase I and PMSF. Lysates were clarified by centrifugation and filtration. Lysates were applied to Ni-NTA (Thermo Scientific HisPur) and washed with a PBS/imidazole gradient. Eluted protein was dialysed overnight at 4 °C into PBS in the presence of His6-ULP1 enzyme with 1 mM dithiothreitol. The dialysed protein was incubated with Ni-NTA beads before concentration to remove uncleaved material, His6-SMT and His6-ULP1. The unbound material was then loaded onto the preparative grade superdex G200 gel filtration column (GE lifesciences) and exchanged into 50 mM Tris pH 8.0, 100 mM NaCl, 1 mM EDTA, and 1 mM dithiothreitol on column. The peak eluting at ~190 ml was concentrated, aliquotted into small volumes, and stored at −80 °C. Surface plasmon resonance studies were carried out with the GE Lifesciences Biacore T100 instrument at 25 °C. STAT5B-WT and N642H variant ligands were thawed and extensively dialysed into HBS-N buffer (GE Lifesciences). Protein samples of 50 μg ml −1 were made by diluting the dialysed stock samples into acetate pH 5.0 buffer immediately before immobilization. Both STAT5B proteins were coupled using EDC/NHS amine coupling chemistry with final immobilization levels of 5345.6 RU for WT and 5433.9 RU for N642H variant. Reference channels received a blank amine coupling protocol. The analyte, phosphopeptide (KAVDG(p)YVKPQI) (Anaspec, Fremont, CA) was prepared by dissolution in water and extensive dialysis into water. The peptide stock solution was stored at 4 °C before analysis. Two-fold dilutions of the phosphopeptide stock were prepared in HBS-EP+ (GE lifesciences) ranging from 100 to 0.78 μM immediately before analysis. Peptide samples were flowed over the immobilized ligand at a rate of 30 μl min −1 with each concentration being run in duplicate. HBS-EP+ was used both as running and regeneration buffer. K D values were calculated using BiaEvaluation software (Biacore AS, Uppsala, Sweeden) by fitting the binding isotherms to a 1:1 Langmuir model. Statistical analysis Two-tailed unpaired t -test was applied using Microsoft Office Excel (Microsoft, Redmond, WA). P <0.05 was considered statistically significant. How to cite this article: Küçük, C. et al . Activating mutations of STAT5B and STAT3 in lymphomas derived from γδ-T or NK cells. Nat. Commun. 6:6025 doi: 10.1038/ncomms7025 (2015). Accession codes. The RNA-Seq and WES sequencing data have been deposited into the SRA database ( http://www.ncbi.nlm.nih.gov/sra ), under the accession code SRA200820 .